Human B cells induce dendritic cell maturation and favour Th2 polarization by inducing OX-40 ligand Dendritic cells (DCs) play a critical role in immune homeostasis by regulating the functions of various immune cells, including T and B cells. Notably, DCs also undergo education on reciprocal signalling by these immune cells and environmental factors. Various reports demonstrated that B cells have profound regulatory functions, although only few reports have explored the regulation of human DCs by B cells. Here we demonstrate that activated but not resting B cells induce maturation of DCs with distinct features to polarize Th2 cells that secrete interleukin (IL)-5, IL-4 and IL-13. B-cell-induced maturation of DCs is contact dependent and implicates signalling of B-cell activation molecules CD69, B-cell-activating factor receptor, and transmembrane activator and calcium-modulating cyclophilin ligand interactor. Mechanistically, differentiation of Th2 cells by B-cell-matured DCs is dependent on OX-40 ligand. Collectively, our results suggest that B cells have the ability to control their own effector functions by enhancing the ability of human DCs to mediate Th2 differentiation. Dendritic cells (DCs) are professional antigen-presenting cells (APCs) and sentinels of the immune system. They perform a prime role in initiating and controlling antigen-specific immune response [1] . These functions of DCs are enabled by their ability to sense and respond to stimuli from their surroundings and to interact with various cells. To perform these functions, DCs transform from an immature state, where they are superior in sensing (antigenic) stimuli, to a mature state, where they are capable of relaying the antigen signatures to adaptive immune cells to induce antigen-specific immune response [1] . DC maturation is characterized by changes in the expression of antigen-presenting molecule HLA-DR, co-stimulatory molecules and cytokine secretion, which influence the outcome of DC interaction with T and B cells [2] . DCs also produce an array of chemokines based on their maturation status to regulate the trafficking of immune cells. In fact, DCs engage in a cross-talk with different immune cells, including T cells, natural killer (NK) cells and B cells. Reciprocal signalling by these cells can regulate the DC maturation and functions. Accordingly, several studies have shown that T and B cells, innate lymphocytes and neutrophils could influence the quality of immune responses elicited by DCs [1] , [3] , [4] , [5] , [6] , [7] , [8] , [9] , [10] , [11] . Activated innate lymphocytes and neutrophils induce maturation of DCs with T helper 1 (Th1) polarizing features [8] , [9] , [10] , [11] . However, education of DCs by T cells reliant on their subsets: regulatory T cells (Tregs) induce tolerogenic feature on DCs, whereas naive and effector memory T cells induce DC maturation with potent T-cell stimulatory capacity [4] , [5] , [6] , [7] . B cells are best known for antibody production. Of note, various reports clearly demonstrated that B cells have profound regulatory functions [3] , [12] , [13] , [14] , [15] , [16] , [17] . However, only few reports have explored the regulation of DC functions by B cells. Murine models have suggested that B cells might favour the induction of non-polarized immune responses by regulating the functions of DCs [18] . Further, a recent study demonstrated that human B cells that receive signalling via CD40 and Toll-like receptor 9 (TLR9) gain the capacity to restrain the maturation and functions of human DCs [19] , although our recent study suggests that regulation of human DCs by B cells depends on the signals they receive [20] . In addition, B cells enhance the production of type I interferon (IFN) by plasmacytoid DCs stimulated with RNA-containing immune complexes [21] . Thus far, only few reports have explored the regulation of human DCs by B cells. Therefore, in the present study we investigated whether B cells could positively regulate human DC maturation and function. We demonstrate that on B-cell receptor (BCR) or CD40-mediated activation, human B cells induce maturation of DCs characterized by enhanced expression of HLA-DR and co-stimulatory molecules CD80, CD86 and CD40. For B cells to exert these effects on DCs, direct cellular contact mediated through molecules associated with B-cell activation such as CD69, B cell-activating factor receptor (BAFF-R) and transmembrane activator and calcium-modulating cyclophilin ligand interactor (TACI) are essential. Further, activated B cells also induce increased secretion of cytokines and selectively modulate the chemokine production of DCs. These B-cell-matured DCs exhibit enhanced CD4 + T cell (Th) stimulatory capacity with unique features to promote Th2 response without affecting other effector Th cell subsets and Tregs. BCR-activated human B cells induce maturation of DCs We first investigated the effect of B cells on phenotype of DCs. Freshly isolated circulating CD19 + B cells, referred as ‘resting B cells’, were cultured with immature DCs for 48 h ( Fig. 1a ). We found that resting B cells do not significantly modify the phenotype of DCs (DC Rest-B ) and the expression of various DC molecules was similar to that of control DCs (DC ctrl ) ( Fig. 1b–d ). These results indicate that in resting phase, B cells do not provide signals to DCs to undergo maturation. Interestingly, when BCR signalling was provided by F(ab′) 2 fragments of anti-human IgM antibodies in the DC–B cell co-culture ( Fig. 1a ), the activated B cells induced maturation of DCs (DC BCR-B ). Thus, DCs showed significantly enhanced expression of co-stimulatory molecules CD80, CD86 and CD40, antigen-presenting molecule HLA-DR and terminal maturation marker CD83 ( Fig. 1b,c ). Consensus with the DC maturation, the expression of antigen uptake receptor CD206 and lipid antigen-presenting molecule CD1a were decreased, whereas the levels of integrin receptor CD11c and C-type lectin receptor DC-SIGN were increased on DC BCR-B ( Fig. 1d ). Similar results were observed with allogenic as well as autologous B cell–DC co-culture, suggesting that the changes in DC phenotype are not due to allogeneic reaction. 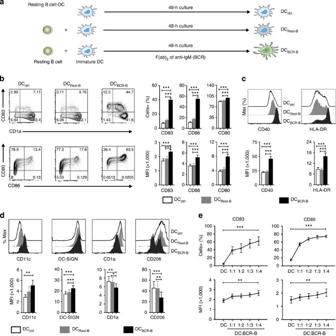Figure 1: BCR-activated B cells induce maturation of DCs. (a) Experimental design. Immature DCs were cultured for 48 h in the medium containing granulocyte macrophage colony-stimulating factor and IL-4 alone (DCctrl), or co-cultured at 1:1 ratio with CD19+B cells that were either in resting phase (DCRest-B) or directly activated in DC–B cell co-culture via BCR stimuli (DCBCR-B). Phenotypic analysis of CD20-negative cells was done by flow cytometry. (b) BCR-activated B cells enhance the expression (% positive cells and mean fluorescence intensity, MFI) of DC activation markers and co-stimulatory molecules. (c) BCR-activated B cells upregulate expression of HLA-DR and CD40 on DCs. (d) Modulation of expression of CD11c, DC-SIGN, CD1a and CD206 on DCs by BCR-activated B cells. Representative plot and mean±s.e.m. of data from 10 to 24 donors. (e) Immature DCs were co-cultured with increasing number of B cells in the presence of BCR stimuli for 48 h and expression (% positive cells and MFI) of CD83 and CD86 was analysed on CD20-negative cells. Mean±s.e.m. of data from four donors. *P<0.05; **P<0.01; ***P<0.001 by one-way analysis of variance test. Figure 1: BCR-activated B cells induce maturation of DCs. ( a ) Experimental design. Immature DCs were cultured for 48 h in the medium containing granulocyte macrophage colony-stimulating factor and IL-4 alone (DC ctrl ), or co-cultured at 1:1 ratio with CD19 + B cells that were either in resting phase (DC Rest-B ) or directly activated in DC–B cell co-culture via BCR stimuli (DC BCR-B ). Phenotypic analysis of CD20-negative cells was done by flow cytometry. ( b ) BCR-activated B cells enhance the expression (% positive cells and mean fluorescence intensity, MFI) of DC activation markers and co-stimulatory molecules. ( c ) BCR-activated B cells upregulate expression of HLA-DR and CD40 on DCs. ( d ) Modulation of expression of CD11c, DC-SIGN, CD1a and CD206 on DCs by BCR-activated B cells. Representative plot and mean±s.e.m. of data from 10 to 24 donors. ( e ) Immature DCs were co-cultured with increasing number of B cells in the presence of BCR stimuli for 48 h and expression (% positive cells and MFI) of CD83 and CD86 was analysed on CD20-negative cells. Mean±s.e.m. of data from four donors. * P <0.05; ** P <0.01; *** P <0.001 by one-way analysis of variance test. Full size image We confirmed that the maturation of DCs was indeed due to signalling by BCR-activated B cells and not due to nonspecific stimulation of DCs by F(ab′) 2 fragments of anti-human IgM antibodies used for the BCR activation of B cells. The phenotype of DCs was unaltered when cultured with F(ab′) 2 fragments of anti-human IgM alone, in the absence of B cells ( Supplementary Fig. 1 ). Further, induction of maturation of DCs by BCR-activated B cells varied directly with the DC:B cell ratio ( Fig. 1e ). Together, these data demonstrate that BCR-mediated activation license human B cells to induce maturation of DCs. Induction of DC maturation by B cells is contact dependent B cells could regulate immune responses both by direct cellular interactions and by secreting various soluble mediators [3] , [12] , [19] . Therefore, we explored the mode of interaction involved in the induction of DC maturation by B cells. The B cells were pre-activated with BCR alone (DC pBCR-B ) or with BCR+CD40-stimulation (DC pBCR+CD40-B ) and immature DCs were co-cultured with these B cells either in direct contact or kept separated in transwells ( Fig. 2a ). In parallel, DCs were also stimulated with supernatant from activated B cells. 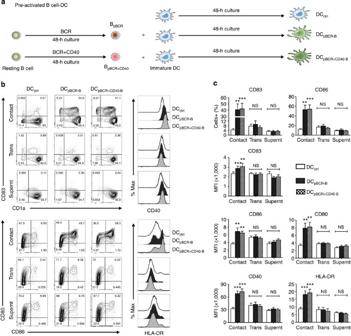Figure 2: Cellular contact is required and sufficient for the induction of maturation of DCs by activated B cells. (a) Pre-activated B cell–DC experimental design. Immature DCs were cultured in medium containing granulocyte macrophage colony-stimulating factor and IL-4 for 48 h either alone (DCctrl) or co-cultured at 1:1 ratio with CD19+B cells that were pre-activated by BCR (DCpBCR-B) or BCR+CD40 (DCpBCR+CD40-B) stimulation. (b,c) DC–B cell co-culture was either done in 96 U-bottomed wells to allow direct contact between DCs and B cells (Contact) or in transwell plate to separate the B cells from DCs (Trans). Immature DCs were also cultured in the supernatants from activated B cells (Supernt). Phenotypic analysis (% positive cells and mean fluorescence intensity, MFI) of DCs that were gated negative for CD20. Representative plot and mean±s.e.m. of data from 7 to 11 donors. (Contact,n=11; Transwell,n=7; Supernatant,n=8). **P<0.01; ***P<0.001; NS, not significant by one-way analysis of variance test. Figure 2: Cellular contact is required and sufficient for the induction of maturation of DCs by activated B cells. ( a ) Pre-activated B cell–DC experimental design. Immature DCs were cultured in medium containing granulocyte macrophage colony-stimulating factor and IL-4 for 48 h either alone (DC ctrl ) or co-cultured at 1:1 ratio with CD19 + B cells that were pre-activated by BCR (DC pBCR-B ) or BCR+CD40 (DC pBCR+CD40-B ) stimulation. ( b , c ) DC–B cell co-culture was either done in 96 U-bottomed wells to allow direct contact between DCs and B cells (Contact) or in transwell plate to separate the B cells from DCs (Trans). Immature DCs were also cultured in the supernatants from activated B cells (Supernt). Phenotypic analysis (% positive cells and mean fluorescence intensity, MFI) of DCs that were gated negative for CD20. Representative plot and mean±s.e.m. of data from 7 to 11 donors. (Contact, n =11; Transwell, n =7; Supernatant, n =8). ** P <0.01; *** P <0.001; NS, not significant by one-way analysis of variance test. Full size image We found that DCs co-cultured in direct contact with activated B cells exhibit phenotypic changes suggestive of maturation, including increased expression of CD83, CD80, CD86, CD40 and HLA-DR ( Fig. 2b,c , panel ‘Contact’). Interestingly, BCR-mediated activation alone appears to be sufficient for B cells to gain capacity to induce maturation of DCs (DC pBCR-B ) as B cells that received additional stimulation via CD40 also induced similar level of maturation of DCs (DC pBCR+CD40-B ) ( Fig. 2b,c ). Furthermore, B cells that received activation signalling via CD40 alone also induced maturation of DCs ( Supplementary Fig. 2 ). Thus, BCR or CD40 signalling enables B cells to induce DC maturation. In contrast to direct contact, when pre-activated B cells were separated from DCs in transwell plates, DC maturation-associated molecules were not upregulated and DCs retained the phenotype similar to control cells (DC ctrl ) ( Fig. 2b,c , panel ‘Trans’). Even soluble mediators present in the supernatants of activated B cells did not promote maturation of DCs ( Fig. 2b,c ; panel ‘Supernt’). Taken together, these results indicated that direct contact with activated B cells is indispensible and sufficient for the induction of maturation of DCs. Of interest, BCR-pre-activated B cells that were paraformaldehyde fixed also induced maturation of DCs, thus suggesting a role for B-cell surface molecules in the process ( Supplementary Fig. 3 ). B-cell activation-associated molecules mediate DC maturation As activation of B cells and contact-dependent interaction between DCs and B cells were necessary for the maturation of DCs, we aimed at identifying the activation-associated B-cell surface molecules implicated in this process. We found that in addition to upregulation of classical B-cell activation-associated molecules, such as HLA-DR, CD25, CD38, CD40, CD80 and CD86, B-cell stimulation also led to significantly enhanced expression of CD69, BAFF-R and TACI ( Fig. 3a,b ). We found that BCR (B BCR ) or BCR+CD40 (B BCR+CD40 ) signalling was superior to CD40 signalling alone in their ability induce the expression of B-cell activation-associated molecules ( Fig. 3a,b ). As CD69, BAFF-R and TACI could interact with corresponding ligands on DCs, we explored the role of these B-cell surface molecules in the process of DC maturation by employing blocking antibodies. 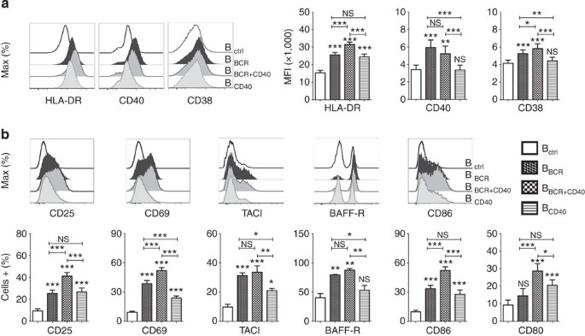Figure 3: Phenotypic analysis of B cells activated with various stimuli. CD19+B cells were either cultured alone (Bctrl) or in the presence of BCR (BBCR) or agonistic CD40 antibody (BCD40) alone, or BCR+CD40 (BBCR+CD40) for 48 h. (a,b) Expression of surface activation markers on B cells as analysed by flow cytometry. Representative plot and mean±s.e.m. of data from five to ten donors. *P<0.05; **P<0.01; ***P<0.001; NS, not significant. Statistical significance as determined by one-way analysis of variance test. Figure 3: Phenotypic analysis of B cells activated with various stimuli. CD19 + B cells were either cultured alone (B ctrl ) or in the presence of BCR (B BCR ) or agonistic CD40 antibody (B CD40 ) alone, or BCR+CD40 (B BCR+CD40 ) for 48 h. ( a , b ) Expression of surface activation markers on B cells as analysed by flow cytometry. Representative plot and mean±s.e.m. of data from five to ten donors. * P <0.05; ** P <0.01; *** P <0.001; NS, not significant. Statistical significance as determined by one-way analysis of variance test. Full size image Interestingly, on blocking TACI, BAFF-R or CD69 individually lead to only minor inhibition of DC maturation. However, blocking all three receptors simultaneously lead to significant inhibition of DC maturation as analysed by the phenotype ( Fig. 4 ). Of note, adhesion molecules CD54 and CD11a/CD18 were found to be not involved in the process. We also found that the expression of CD69 on B cells implicates BCR or CD40 signals received by the B cells but not feedback signals by BAFF as treatment of B cells with BAFF led to only minor changes in the expression of CD69 on B cells. 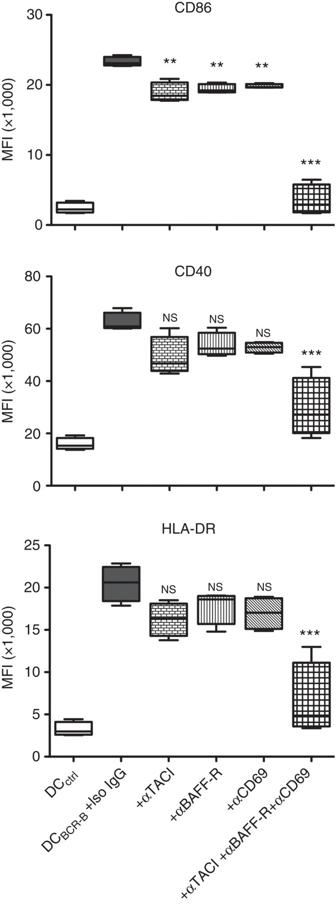Figure 4: Several surface molecules on activated B cells are involved in contact-dependent induction of maturation of DCs. Immature DCs were cultured in medium containing granulocyte macrophage colony-stimulating factor and IL-4 for 48 h either alone (DCctrl), or co-cultured at the ratio of 1:1 with CD19+B cells in the presence of BCR stimuli. Co-culture was done either in the presence of isotype control mouse IgG (DCBCR-B+Iso IgG) or blocking antibodies to TACI (+αTACI), BAFF-R (+αBAFF-R), CD69 (+αCD69) alone or together (+αTACI+αBAFF-R+αCD69). Flow cytometric analysis of phenotype (mean fluorescence intensity, MFI) of CD20-negative DC population was performed. Mean±s.e.m. of data from four donors. **P<0.01; ***P<0.001; NS, not significant by one-way analysis of variance test. Figure 4: Several surface molecules on activated B cells are involved in contact-dependent induction of maturation of DCs. Immature DCs were cultured in medium containing granulocyte macrophage colony-stimulating factor and IL-4 for 48 h either alone (DC ctrl ), or co-cultured at the ratio of 1:1 with CD19 + B cells in the presence of BCR stimuli. Co-culture was done either in the presence of isotype control mouse IgG (DC BCR-B +Iso IgG) or blocking antibodies to TACI (+αTACI), BAFF-R (+αBAFF-R), CD69 (+αCD69) alone or together (+αTACI+αBAFF-R+αCD69). Flow cytometric analysis of phenotype (mean fluorescence intensity, MFI) of CD20-negative DC population was performed. Mean±s.e.m. of data from four donors. ** P <0.01; *** P <0.001; NS, not significant by one-way analysis of variance test. Full size image Modulation of DC cytokines and chemokines by activated B cells During the process of maturation, in addition to upregulation of expression of surface markers, DCs also secrete increased amount of various cytokines and chemokines that play a critical role in creating inflammation, polarization of T cells and migration of diverse immune cells. Analysis of supernatants from DC–B cell co-cultures showed that in the presence of resting B cells (DC Rest-B ) only marginal changes in the cytokine profile were observed ( Fig. 5a ). When B cells were activated directly in the DC–B cell co-culture via BCR signalling (DC BCR-B ), B cells stimulated DCs to produce significant amount of IL-6, tumour necrosis factor (TNF)-α and IL-10 ( Fig. 5a ). Similarly, co-culture of DCs in direct contact with B cells that were pre-activated with either BCR alone (DC pBCR-B ) or BCR+CD40 (DC pBCR+CD40-B ) significantly enhanced the production of above cytokines ( Fig. 5b ). However, DC co-cultured with pre-activated B cells in transwell culture system did not produce increased amount of cytokines. As the above cytokines in the co-culture could be derived from DCs as well as B cells, we wanted to confirm that increased secretion of cytokines in DC–B cell co-culture was mainly because of DCs. In fact, intracellular staining showed that activated B cells induced significantly increased frequency of IL-6- and TNF-α-producing DCs ( Fig. 5c ), suggesting that increased cytokine levels in DC–B cell co-culture were mainly contributed from DCs. 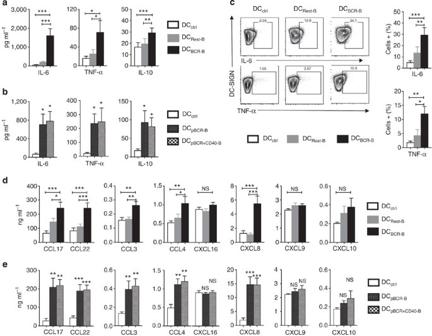Figure 5: Effect of activated B cells on the secretion of cytokines and chemokines by DCs. Immature DCs were cultured for 48 h in the medium containing granulocyte macrophage colony-stimulating factor and IL-4 alone (DCctrl), or co-cultured at 1:1 ratio with CD19+B cells that were either in resting phase (DCRest-B) or directly activated in DC-B cell co-culture via BCR stimuli (DCBCR-B). Alternatively, DCs were also co-cultured with CD19+B cells that were pre-activated by BCR (DCpre-BCR-B) or BCR+CD40 (DCpre-BCR+CD40-B) stimulation for 48 h. (a,b) Supernatants of co-cultures were analysed for the amounts (pg ml−1) of cytokines. Mean±s.e.m. of data from ten donors. (c) CD20-negative DCs from B cell–DC co-cultures were analysed for the intracellular expression of IL-6 and TNF-α by flow cytometry. Representative plot and mean±s.e.m. of data from four donors. (d,e) Amount of chemokines in the culture supernatants of DC–B cell co-cultures. Mean±s.e.m. of data from ten donors. *P<0.05; **P<0.01; ***P<0.001; NS, not significant by one-way analysis of variance test. Figure 5: Effect of activated B cells on the secretion of cytokines and chemokines by DCs. Immature DCs were cultured for 48 h in the medium containing granulocyte macrophage colony-stimulating factor and IL-4 alone (DC ctrl ), or co-cultured at 1:1 ratio with CD19 + B cells that were either in resting phase (DC Rest-B ) or directly activated in DC-B cell co-culture via BCR stimuli (DC BCR-B ). Alternatively, DCs were also co-cultured with CD19 + B cells that were pre-activated by BCR (DC pre-BCR-B ) or BCR+CD40 (DC pre-BCR+CD40-B ) stimulation for 48 h. ( a , b ) Supernatants of co-cultures were analysed for the amounts (pg ml −1 ) of cytokines. Mean±s.e.m. of data from ten donors. ( c ) CD20-negative DCs from B cell–DC co-cultures were analysed for the intracellular expression of IL-6 and TNF-α by flow cytometry. Representative plot and mean±s.e.m. of data from four donors. ( d , e ) Amount of chemokines in the culture supernatants of DC–B cell co-cultures. Mean±s.e.m. of data from ten donors. * P <0.05; ** P <0.01; *** P <0.001; NS, not significant by one-way analysis of variance test. Full size image Next, we analysed the supernatant of B cell–DC co-culture for various chemokines that could influence the trafficking of immune cells. Similar to cytokine profiles, irrespective of B-cell activation method, that is, B cells activated directly in the DC:B cell co-cultures via BCR signalling (DC BCR-B ) ( Fig. 5d ) or pre-activated with BCR (DC pBCR-B ), or with BCR+CD40 (DC pBCR+CD40-B ) before co-culture with DCs ( Fig. 5e ), stimulated DCs to produce significantly increased amounts of CCL17 and CCL22 (ligands for CCR4), CCL3 and CCL4 (ligands for CCR5), and CXCL8 (IL-8, ligand for CXCR1 and CXCR2). In contrast, CXCL16 (ligand of CXCR6), and CXCL9 and CXCL10 (ligands for CXCR3), were not significantly altered ( Fig. 5d,e ). To explore the contribution of DCs to the chemokines in the B cell–DC co-culture, we analysed the supernatants of activated B cells. On BCR (B BCR ) or BCR+CD40 (B BCR+CD40 )-mediated activation, B cells did not secrete CCL17, CCL22 and CXCL16, indicating that these chemokines in DC–B cell co-cultures were contributed mainly by DCs. However, the secretion of CCL3, CCL4, CXCL9 and CXCL10 by activated B cells was either on par with those levels observed in DC–B cell co-cultures or even higher, suggesting that these chemokines in DC–B cell co-cultures were contributed mainly by B cells rather than DCs ( Supplementary Fig. 4a ). Furthermore, analysis of intracellular expression of chemokines in DCs revealed that activated B cells enhanced the frequency of CXCL8-producing DCs, but not CCL4 ( Supplementary Fig. 4b ). Together, these findings provide a pointer towards selective induction of DC chemokines by activated B cells. T-cell stimulation and polarization by B-cell-matured DCs DCs matured under the influence of B cells were evaluated for T-cell stimulatory capacity by co-culturing B-cell-depleted DCs with CD4 + T cells (Th cells) ( Fig. 6a ). Corroborating the DC phenotype and cytokine profile, resting B cells did not alter the capacity of DCs (DC Rest-B ) to induce T-cell proliferation and was similar to control DCs (DC ctrl ). On the contrary, DCs that were ‘educated’ by activated B cells (DC BCR-B ) stimulated significant proliferation of T cells ( Fig. 6b ) and was associated with significant production of T-cell-derived cytokine IL-2 ( Fig. 6c ). Further, our results also indicated that DCs that received maturation signals from B cells pre-activated with either BCR alone (DC pBCR-B ) or with BCR+CD40-stimulation (DC pBCR+CD40-B ) were similar in their ability to stimulate T-cell proliferation and to induce IL-2 in proliferating T cells ( Supplementary Fig. 5a ). On the contrary, DCs cultured either in transwell plates ( Supplementary Fig. 5b ) or with supernatants of activated B cells ( Supplementary Fig. 5c ) did not promote T-cell proliferation and IL-2 secretion, thus further confirming the indispensability of cellular contact between DCs–B cells for the functional maturation of DC. 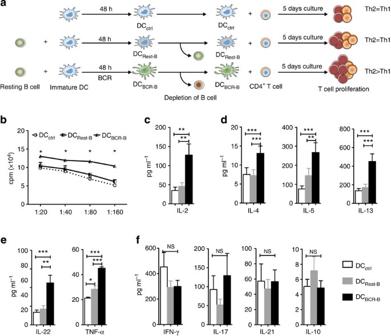Figure 6: B-cell-matured DCs induce proliferation of CD4+T cells producing increased amounts of Th2 type cytokines. (a) Experimental design. Immature DCs were cultured for 48 h in the medium containing granulocyte macrophage colony-stimulating factor and IL-4 alone (DCctrl, or co-cultured at 1:1 ratio with CD19+B cells that were either in resting phase (DCRest-B) or directly activated in DC-B cell co-culture via BCR stimuli (DCBCR-B). DCs were purified from B cell–DC co-culture by depleting B cells using CD20 microbeads. CD4+T cells were co-cultured with DC at various ratios for 4 days. (b) DC-mediated CD4+T-cell proliferation as determined by [3H] incorporation assay. Values are presented as counts per minute (cpm). Data are mean±s.e.m. from quadruplicate wells and representative of five independent experiments. (c–f). Supernatants from DC–T cell co-cultures at 1:20 ratio were analysed for different T-cell cytokines. Mean±s.e.m. of data from eight to ten donors. *P<0.05; **P<0.01; ***P<0.001; NS, not significant by one-way analysis of variance test. Figure 6: B-cell-matured DCs induce proliferation of CD4 + T cells producing increased amounts of Th2 type cytokines. ( a ) Experimental design. Immature DCs were cultured for 48 h in the medium containing granulocyte macrophage colony-stimulating factor and IL-4 alone (DC ctrl , or co-cultured at 1:1 ratio with CD19 + B cells that were either in resting phase (DC Rest-B ) or directly activated in DC-B cell co-culture via BCR stimuli (DC BCR-B ). DCs were purified from B cell–DC co-culture by depleting B cells using CD20 microbeads. CD4 + T cells were co-cultured with DC at various ratios for 4 days. ( b ) DC-mediated CD4 + T-cell proliferation as determined by [ 3 H] incorporation assay. Values are presented as counts per minute (cpm). Data are mean±s.e.m. from quadruplicate wells and representative of five independent experiments. ( c – f ). Supernatants from DC–T cell co-cultures at 1:20 ratio were analysed for different T-cell cytokines. Mean±s.e.m. of data from eight to ten donors. * P <0.05; ** P <0.01; *** P <0.001; NS, not significant by one-way analysis of variance test. Full size image To further understand the influence of B-cell-matured DCs on CD4 + T-cell responses, we measured the levels of various Th cell cytokines in the DC–T cell supernatants. Interestingly, DC BCR-B skewed Th-cell responses towards Th2 as indicated by significant secretion of Th2 cell cytokines, including IL-4, IL-5 and IL-13 ( Fig. 6d ). In addition, modest increase in TNF-α and IL-22 was also observed ( Fig. 6e ). However, IFN-γ, signature cytokine of Th1 and IL-17, signature cytokine of Th17, and also IL-21 and IL-10 were not altered ( Fig. 6f ). B-cell-matured DCs selectively induce Th2 differentiation Next we investigated the ability of B-cell-matured DCs to modulate the differentiation of naive Th cells. We found that DCs that received signals from BCR-activated B cells (DC BCR-B ) significantly increased the frequencies of Ki-67 + and IL-2 + T cells (T BCR-B-DC ) ( Fig. 7a,b ), indicating enhanced proliferation of naive T cells. However, frequencies of Ki-67 + and IL-2 + T cells were not significantly altered when naive Th cells were co-cultured with DCs that received signals from resting B cells (T Rest-B-DC ). Moreover, naive T cells cultured with DC BCR-B significantly downregulated the expression of CD27 and CCR7 compared with T cells cultured with DC ctrl or DC Rest-B ( Fig. 7c,d ). These results suggested that B-cell-matured DCs induce proliferation and differentiation of effector T cells. 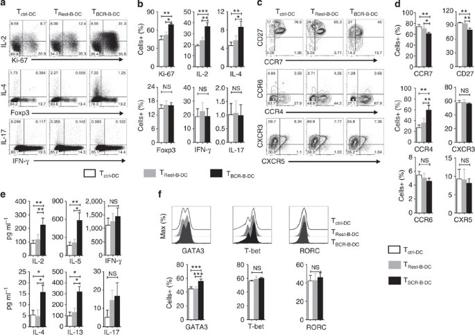Figure 7: B cell-matured DCs favour polarization of naive CD4+T cells to Th2 cells. Immature DCs were cultured for 48 h in the medium containing granulocyte macrophage colony-stimulating factor and IL-4 alone (DCctrl), or co-cultured at 1:1 ratio with CD19+B cells that were either in resting phase (DCRest-B) or directly activated in DC–B cell co-culture via BCR stimuli (DCBCR-B). DCs were purified from B cell–DC co-culture by depleting B cells. CD4+CD45RO−naive Th cells were co-cultured with control DCs (Tctrl-DC) or activated B-cell-matured DCs (TBCR-B-DC) or resting B-cell-stimulated DC (TRest-B-DC) at the ratio of 20:1 for 6 days. (a,b) CD3+T cells were analysed for the intracellular expression of cytokines and transcription factors by flow cytometry. Representative plot and mean±s.e.m. of data from ten donors. (c,d) CD3+T cells were analysed for the surface phenotype by flow cytometry. Representative plot and mean±s.e.m. of data from five donors. (e) After 6 days, supernatants from DC–T cell co-cultures were analysed for various T-cell cytokines. Mean±s.e.m. of data from eight to ten donors. (f) CD3+T cells were analysed for intracellular expression of transcription factors by flow cytometry. Representative plot and mean±s.e.m. of data from four donors. *P<0.05; **P<0.01; ***P<0.001; NS, not significant by one-way analysis of variance test. Figure 7: B cell-matured DCs favour polarization of naive CD4 + T cells to Th2 cells. Immature DCs were cultured for 48 h in the medium containing granulocyte macrophage colony-stimulating factor and IL-4 alone (DC ctrl ), or co-cultured at 1:1 ratio with CD19 + B cells that were either in resting phase (DC Rest-B ) or directly activated in DC–B cell co-culture via BCR stimuli (DC BCR-B ). DCs were purified from B cell–DC co-culture by depleting B cells. CD4 + CD45RO − naive Th cells were co-cultured with control DCs (T ctrl-DC ) or activated B-cell-matured DCs (T BCR-B-DC ) or resting B-cell-stimulated DC (T Rest-B-DC ) at the ratio of 20:1 for 6 days. ( a , b ) CD3 + T cells were analysed for the intracellular expression of cytokines and transcription factors by flow cytometry. Representative plot and mean±s.e.m. of data from ten donors. ( c , d ) CD3 + T cells were analysed for the surface phenotype by flow cytometry. Representative plot and mean±s.e.m. of data from five donors. ( e ) After 6 days, supernatants from DC–T cell co-cultures were analysed for various T-cell cytokines. Mean±s.e.m. of data from eight to ten donors. ( f ) CD3 + T cells were analysed for intracellular expression of transcription factors by flow cytometry. Representative plot and mean±s.e.m. of data from four donors. * P <0.05; ** P <0.01; *** P <0.001; NS, not significant by one-way analysis of variance test. Full size image Of note, CCR7 − CD27 − T cells were previously shown to contain mainly the IL-4-producing T cells [22] . In line with this report, we further found that DC BCR-B significantly increased the frequency of CCR4 + T cells but did not alter the expression of CXCR3, CXCR5 and CCR6 on T cells ( Fig. 7c,d ). Of particular relevance, CCR4 has been shown to be preferentially expressed on Th2 cells and Tregs [23] . Interestingly, we found that DC BCR-B significantly increased the frequency of IL-4-expressing cells but not FoxP3 + cells ( Fig. 7a,b ). Thus, our findings suggest that B-cell-matured DCs selectively induce differentiation of Th cells towards Th2 phenotype and not Tregs. However, the frequency of IFN-γ-expressing Th1 cells and IL-17-secreting Th17 cells was unaltered by DC BCR-B ( Fig. 7a,b ). Further, analysis of the supernatants for T-cell cytokines revealed that DC BCR-B significantly increased the secretion of IL-2, which supports the proliferating T cells ( Fig. 7e ). Interestingly, these T cells (T BCR-B-DC ) secreted significantly higher amount of Th2 cytokines such as IL-4, IL-5 and IL-13 ( Fig. 7e ). However, the secretion of IFN-γ and IL-17 by T cells was not significantly altered by DC BCR-B ( Fig. 7e ). Finally, we examined the expression of Th cell subset-specific transcription factors to substantiate the surface phenotype and cytokine profile data of T cells. DC BCR-B significantly enhanced the expression GATA3, the master regulator of Th2 cells ( Fig. 7f ) [24] , while the expression of T-bet (Th1), RORC (Th17) and Foxp3 (Tregs) was not altered by DC BCR-B ( Fig. 7a,b,f ). Of note, DCs activated by B cells pre-stimulated with BCR (DC pBCR-B ) or CD40 alone (DC pCD40-B ), or BCR+CD40 (DC pBCR+CD40-B ), were also capable of inducing naive Th-cell activation, proliferation and differentiation to Th2 phenotype to a similar extent ( Supplementary Fig. 6 ). Taken together, our results demonstrate that DCs that receive signals from activated B cells selectively induce differentiation of Th2 cells from naive T cells. Th2 polarization by B-cell-matured DCs is OX-40 ligand-dependent We explored the mechanism of induction of Th2 cells by B-cell-matured DCs. We observed that activated B cells did not induce Th1-triggerring molecules in DCs such as IL-12 and CD70 ( Fig. 8a,c ), which is in consensus with the unaltered IFN-γ-expressing cells and IFN-γ secretion by T cells that were stimulated by B-cell-matured DCs. Further, B cells did not stimulate the production of IL-33 in DCs, a cytokine that was shown to amplify both Th1- and Th2-type responses in humans ( Fig. 8b ) [25] . 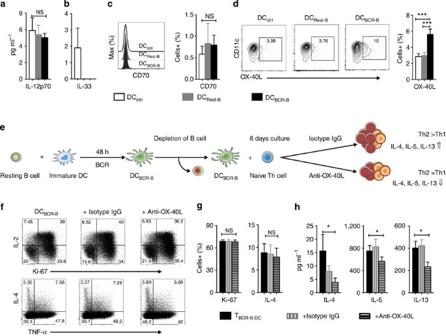Figure 8: Th2 polarization by B-cell-matured DCs is dependent in part on OX-40 ligand. Immature DCs were cultured for 48 h in the medium containing granulocyte macrophage colony-stimulating factor and IL-4 alone (DCctrl), or co-cultured at 1:1 ratio with CD19+B cells that were either in resting phase (DCRest-B) or directly activated in DC–B cell co-culture via BCR stimuli (DCBCR-B). (a,b) Supernatants of DC–B cell co-cultures were analysed for IL-12p70 and IL-33. Mean±s.e.m. of data from five to ten donors. (c,d) Expression of CD70 and OX-40L on DCs that were gated negative for CD20. Representative plot and mean±s.e.m. of data from ten donors. (e) Experimental design for OX-40L blocking experiments and repercussion on T-cell cytokines. B-cell-matured DCs were purified from the DC–B cell co-cultures by depleting B cells. CD4+CD45RO−naive Th cells were co-cultured with these B-cell-matured DC at the ratio of 20:1 for 6 days (TBCR-B-DC) either alone or in the presence of isotype IgG antibody (+Isotype IgG) or blocking antibody to OX-40L +Anti-OX-40 L). (f,g) CD3+T cells were analysed for intracellular expression of cytokines or Ki-67 by flow cytometry and (h) supernatants from DC–T cell co-cultures were analysed for different T-cell cytokines. Representative plot and mean±s.e.m. of data from five donors. *P<0.05; ***P<0.001 NS, not significant by one-way analysis of variance test. Figure 8: Th2 polarization by B-cell-matured DCs is dependent in part on OX-40 ligand. Immature DCs were cultured for 48 h in the medium containing granulocyte macrophage colony-stimulating factor and IL-4 alone (DC ctrl ), or co-cultured at 1:1 ratio with CD19 + B cells that were either in resting phase (DC Rest-B ) or directly activated in DC–B cell co-culture via BCR stimuli (DC BCR-B ). ( a , b ) Supernatants of DC–B cell co-cultures were analysed for IL-12p70 and IL-33. Mean±s.e.m. of data from five to ten donors. ( c , d ) Expression of CD70 and OX-40L on DCs that were gated negative for CD20. Representative plot and mean±s.e.m. of data from ten donors. ( e ) Experimental design for OX-40L blocking experiments and repercussion on T-cell cytokines. B-cell-matured DCs were purified from the DC–B cell co-cultures by depleting B cells. CD4 + CD45RO − naive Th cells were co-cultured with these B-cell-matured DC at the ratio of 20:1 for 6 days (T BCR-B-DC ) either alone or in the presence of isotype IgG antibody (+Isotype IgG) or blocking antibody to OX-40L +Anti-OX-40 L). ( f , g ) CD3 + T cells were analysed for intracellular expression of cytokines or Ki-67 by flow cytometry and ( h ) supernatants from DC–T cell co-cultures were analysed for different T-cell cytokines. Representative plot and mean±s.e.m. of data from five donors. * P <0.05; *** P <0.001 NS, not significant by one-way analysis of variance test. Full size image As DCs did not produce Th2-promoting cytokines, we next investigated the expression of Th2-inducing surface molecules on DCs. Interestingly, we found that activated B cells, but not resting B cells, significantly upregulated the expression of OX-40 ligand (OX-40L) on DCs ( Fig. 8d ). Thus, upregulation of OX-40L in the absence of IL-12 and CD70 expression on B-cell-matured DCs suggested that its interaction with OX-40 on T cells is responsible for driving Th2 polarization. Of particular relevance, epithelial cell-derived thymic stromal lymphopoietin (TSLP) was also shown to upregulate the expression of OX-40L on DCs and is implicated in Th2 responses during allergy reactions [26] . Hence, we compared the phenotype and T-cell-stimulating abilities of TSLP-treated DCs (DC TSLP ) and B-cell-matured DCs (DC pBCR-B ). Surprisingly, with the exception of CD86, TSLP did not significantly upregulate the activation-associated molecules on DCs and DC TSLP failed to induce significant T-cell proliferation, as compared with DC pBCR-B ( Supplementary Fig. 7a,b,d ). Interestingly, although the expression of GATA3 was enhanced only by DC pBCR-B , both DC TSLP as well as DC pBCR-B enhanced the production of Th2 cytokines, IL-5 and IL-13 to a similar extent, without modifying IFN-γ secretion ( Supplementary Fig. 7e,f ). Consistent with this observation, induction of OX-40L expression on DCs by BCR- or CD40-activated B cells was similar to that of TSLP signalling ( Supplementary Fig. 7c ). These findings further support that B-cell-matured DC-induced Th2 polarization involves OX-40L. To confirm this, blocking antibodies to OX-40L were employed in the co-culture of naive T cells and DC BCR-B ( Fig. 8e ). Following 6 days of culture, the frequencies of Ki-67 + and IL-2 + T cells in the presence of anti-OX-40L antibodies were similar to isotype antibodies ( Fig. 8f,g ), suggesting that blocking OX-40L did not interfere with DC-induced proliferation and survival of naive T cells. Although blocking of OX-40L did not inhibit the frequency of IL-4-expressing T cells ( Fig. 8f,g ), there was significant decrease in the amount of secretion of Th2 cytokines, IL-4, IL-5 and IL-13 ( Fig. 8h ). Together, our results demonstrate that Th2 differentiation by B-cell-matured DCs is dependent at least in part on OX-40 ligand. Th2 cells induced by B-cell-matured DCs promote IgE production To further evaluate the physiological role of Th2 polarization induced by B-cell-matured DCs, we co-cultured the differentiated T cells with freshly isolated B cells and determined their ability to induce IgE production ( Supplementary Fig. 8a ). Preliminary results revealed that Th2 cells induced by B-cell-matured DCs are capable of stimulating B cells to produce IgE, which was similar to that of T cells activated by TSLP–DC ( Supplementary Fig. 8b ). However, the levels of IgE induced by these Th2 cells were low and variable, and more studies with additional donors are required to provide fully conclusive results. Of much importance in recent advances in B-cell biology, IL-10-secreting regulatory B cells are claimed to restrain the inflammatory responses by inhibiting proinflammatory cytokines, Th1/Th17 cell development and by facilitating Treg differentiation [12] , [15] , [27] , [28] . In addition, B-cell gene therapy approach has been exploited for the induction of antigen-specific immune tolerance [29] . However, pathogenic role of B cells by the way of T-cell stimulation or via autoantibodies is well documented in autoimmune and inflammatory diseases [30] , [31] , [32] , [33] . Thus, B cells exert both effector and regulatory functions in co-ordination with T cells and DCs during antigen-specific response. Our results demonstrate that B cells when activated, but not at resting phase, induce maturation of DCs with distinct features to polarize T cells. In consensus with our report, previous studies have also shown that human DC maturation could be induced on interaction with activated immune cells, but not with resting cells, wherein naive and effector T cells, IL-2-activated NK cells, antigen-activated NKT cells and γδ T cells, and also TLR-stimulated neutrophils induce maturation of DCs and increase their T-cell stimulatory capacity [1] , [3] , [7] , [8] , [9] , [10] . Several reports have demonstrated that B cells have the capacity to regulate the various facets of DC functions both in vitro and in vivo , to coordinate the process of immune response. B-cell-derived cytokines and chemokines play an important role in the migration of DC subsets. By guiding the expression of CXCL13 on lymphotoxin β-receptor-expressing follicular stromal cells in the spleen, B cell-derived membrane lymphotoxin has been demonstrated to synchronize the migration of a CXCR5 + CD11c + subset of murine DCs for the development of IL-4-producing Th2 cells [34] , [35] . By binding to CD4, IL-16, a polypeptide cytokine secreted by B cells, could induce migration of circulating human CD4 + CD11c + blood DC subset [36] . As IL-16 could also induce migration of CD4 + T cells, B cells might mediate cross-talk between DC-CD4 + T cells–B cells. In addition, via production of antibodies, B cells are also known to regulate DC maturation, activation and functions by engaging Fc receptors or non-Fc receptors, such as CD40, or C-type lectin receptors and T-cell activation [3] , [37] , [38] , [39] , [40] , [41] , [42] , [43] . A previous study in B-cell-deficient mice has indicated that B cells might affect the Th1/Th2 cytokine balance by regulating the function of DCs [18] . The authors found that DCs from B-cell-deficient μMT mice that were injected with keyhole limpet haemocyanin emulsified in complete Freund’s adjuvant, induced differentiation of CD4 + T cells that secreted IL-2, IFN-γ, IL-5 and IL-10. However, unlike DCs from wild-type mice, they failed to induce IL-4. Mechanistically, as compared with DCs from wild-type mice, DCs from μMT mice produced higher levels of IL-12 when pulsed with keyhole limpet haemocyanin. This report suggested that B-cell-derived IL-10 might regulate the production of IL-12 by DCs and consequently Th1/Th2 cytokine response. Similarly, DCs from B-cell-deficient mice infected with Candida albicans and Aspergillus fumigatus also produced higher quantities of IL-12 and lower amounts of IL-10 that might favour enhanced Th1 responses observed in these mice [44] . In line with these reports, B-cell-derived IL-10 was found to be critical for favouring Th2 polarization in Leishmania infection model in mice by downregulating IL-12 production by DCs [45] . However, in our study and in another report, CD19 + peripheral human B cells, when activated through BCR alone or with CD40, did not produce significant amounts of IL-10 (ref. 16 ). These results thus indicated that B cells could regulate DC cytokines and T-cell polarization both via cytokine-dependent (similar to IL-10) and -independent manner (as described in this report), depending on the context of immune response or possibly depending on the particular subset of B cells. Morva et al. [19] recently reported that B cells that received activation signalling via combination of TLR9 (CpG) and CD40 restrain the maturation and function of human DCs. It is known that TLR9 signalling in combination with BCR stimulation or CD40-mediated activation renders human B cells to gain regulatory properties [12] , [15] , [16] . In addition, B cells that receive signals only through TLR9 could also regulate the differentiation and function of DCs [46] , [47] . All these results suggest that regulatory B cells could suppress the differentiation, maturation and function of DCs, and consequently could play a role in immune tolerance and in preventing inflammatory responses similar to those reported in the case of Tregs. However, our recent results also suggested that the repercussion of DC–B cell cross-talk on DC functions might depend on the type of activation signals received by B cells [20] , wherein we found that B cells that received activation signals via BCR alone were not capable of blocking the differentiation of monocyte-derived DCs and did not inhibit TLR-mediated maturation of DCs. These findings are supported by previous reports that have revealed that based on the activation status, B cells might exert either tolerogenic or stimulatory effects on immune cells [48] , [49] . Here we show that B cells pre-activated with either BCR or CD40 stimulation, or both, are capable of inducing maturation of DCs. Further, we found that contact-dependent interaction mediated by B-cell activation-associated molecules such as CD69, BAFF-R and TACI is involved in DC maturation. Interestingly, several studies have shown that activation-associated molecules of T cells and NKT cells, such as CD69 and CD40L, could modulate maturation and function of APCs, including DCs, monocytes and macrophages [50] , [51] . CD69 is shown to be involved in the regulation of sphingosine 1-phosphate receptor-1-mediated DC migration into lymph nodes and lymphocyte egress from lymph nodes [52] . Although till date the receptor binding to CD69 is elusive, it could be speculated that B cells on receiving activation signals, upregulate CD69, which interacts with surface receptor on DCs to induce activation. However, more studies are needed to clarify the role of CD69 in B-cell-mediated regulation of DC maturation and function. Interaction of TACI on B cells with membrane-bound BLys (B-lymphocyte stimulator)/BAFF on DCs was shown to be important for priming naive CD8 + T cells in vivo [53] , thus supporting our findings on the role of TACI and BAFF-R in DC activation. Notably, despite lower expression of these activation molecules, B cells stimulated with CD40 or CD40L+IL-4 induced DC maturation similar to BCR signalling ( Supplementary Fig. 9 ). Interestingly, although activated naive (CD27 - CD19 + ) as well as memory (CD27 + CD19 + ) B cells were capable of inducing DC activation, our preliminary results indicate that naive B cells, but not memory B cells, require both BCR as well as CD40 signalling to be able to induce DC maturation. Based on these findings we believe that in addition to TACI, BAFF-R and CD69, other B-cell surface molecules, yet to be identified, are also required for the induction of DC maturation by activated B cells. Activated T cells, innate lymphocytes and neutrophils have been shown to induce maturation of DCs with Th1 cell polarization. Further, Th1 polarization was found to be due to enhanced secretion of IL-12p70 by DCs, which is facilitated at least in part by IFN-γ secretion, in case of T and NK cells, and by TNF-α production in case of neutrophils [8] , [9] , [10] , [11] . On the other hand, in our study, we found that B-cell-matured DCs did not display significant amount of Th1-inducing molecules such as IL-12p70 and CD70, which explains the unchanged Th1 differentiation. Similarly, lack of specific polarizing cytokines could be the possible reason for B-cell-matured DCs not to favour the differentiation of Th17 cells (IL-1β), follicular Th (Tfh) cells (IL-12 and IL-21) and Tregs (TGF-β). However, B-cell-matured DCs secreted moderate amount of IL-6 and TNF-α, which are the polarizing cytokines for human Th22 (ref. 54 ). These cytokines could be responsible for the moderate increase in IL-22 expression in T cells by B-cell-matured DCs. Development of Th2 cells is facilitated by various cytokines, such as IL-4, TSLP and IL-33, in the absence of IFN-γ and IL-12 signalling [26] , [55] , [56] . It is well known that DCs do not contribute to Th2 polarization by secreting IL-4. However, T-cell stimulation by DCs in the presence of IL-4 contributed by other immune cells such as basophils, mast cells, eosinophils and naive CD4 + T cells could support Th2 differentiation [55] . DCs could also induce IL-4 production from some of these cells via IL-33. It was demonstrated that IL-33 acts on mast cells via ST2 and activates nuclear factor-κB and mitogen-activated protein kinase [57] . Alternatively, IL-33 could directly initiate the production of Th2 cytokines from polarized Th2 cells in vitro and promote IL-4, IL-5 and IL-13 in vivo [57] . However, we could not detect IL-33 in the culture supernatant of B-cell-matured DCs, thus ruling out a role for IL-33-mediated Th2 polarization by B-cell-matured DCs. In addition to cytokines, signalling mediated by interaction of OX-40L, one of the members of the TNF receptor superfamily molecules on DCs, with OX-40 on T cells could also favour Th2 cell responses [58] , [59] , [60] , [61] , [62] . DCs do not express OX40L constitutively, rather expression of which is induced when cells sense activation signals from antigens. Similarly, naive CD4 + T cells lack the expression of OX-40 and is transiently induced on these cells when they receive activation signals from APCs [63] . We found that along with other co-stimulatory molecules of B7 family, activated B cells significantly upregulated the expression of OX-40L on DCs, which was similar to TSLP–DC. The interaction of these B7 co-stimulatory molecules with CD28 on T cells could sustain the expression of OX-40 on T cells [63] . Of note, blocking OX-40L on DCs significantly inhibited the secretion of Th2 cytokines IL-4, IL-5 and IL-13. Our results thus demonstrate that B-cell-matured DCs could induce Th2 response at least in part through OX-40L. Interestingly, DC-produced IL-6 was also shown to promote Th2 differentiation by inducing STAT3-mediated c-Maf and NFATc2 expression [64] , [65] , [66] , [67] , and could interfere with development of Th1 cells by upregulating suppressor of cytokine signalling 1 expression [68] . In this context, in addition to OX-40L, IL-6 produced by B-cell-matured DCs might also be involved in the induction of Th2 cells. We also show that Th2 cells differentiated by B-cell-matured DCs are capable of stimulating IgE production in B cells, similar to TSLP–DC-activated T cells. In fact, previous studies have shown that IL-4 and IL-13 secreted by Th2 cells mediate IgE responses from B cells [69] , [70] . Therefore, based on these reports, it is likely to be that IL-4 and/or IL-13, secreted by Th2 cells that were differentiated by B-cell-matured DCs, are involved in the production of IgE from B cells. However, further investigations are required to confirm these preliminary results. In summary, our results indicate that B cells have the ability to control their own effector functions by enhancing Th2-differention ability of human DCs. However, promotion of Th2 polarization by B cells via DCs might act as double-edged sword. In case of infection, differentiated Th2 cells might support the production of antibodies from B cells and to neutralize the pathogens and their derived products. Conversely, in autoimmune and allergic diseases, Th2 cells that were polarized by B-cell-matured DCs could amplify autoimmune/inflammatory responses by providing help for autoantibody/IgE-producing B cells. Further, by enhancing the production of chemokines CCL17 and CCL22 in DCs, activated B cells might also promote recruitment of Th2 cells. CCL17 and CCL22 are known to recruit CCR4 + Tregs as well and are expected to act as inflammation-limiting factor in the initial phase of immune response. However, it is well established that Tregs are incompetent to regulate sustained chronic inflammation. Under such inflammatory conditions as in the case of lupus, stimulation of B-cell-derived IL-10 production by CpG-DNA and activation of regulatory B cells could act as inflammation-limiting factor by suppressing the BCR/CD40-activated B-cell-mediated maturation of DCs. Reagents and antibodies The medium used throughout was RPMI 1640 supplemented with 10% (vol/vol) heat-inactivated (56 °C, 30 min) FCS, 100 U ml −1 penicillin and 100 μg ml −1 streptomycin. F(ab′) 2 fragments of affinity-purified goat anti-human IgM (Fc fragment-specific) was obtained from Jackson ImmunoResearch Laboratories (West Grove, USA). Cell purification reagents such as microbeads and isolation kits were from Miltenyi Biotec (Paris, France). Purification of cells Peripheral blood mononuclear cells (PBMCs) were obtained from buffy bags of healthy donors by Ficoll density gradient centrifugation. Buffy bags of the healthy blood donors were purchased from Centre Necker-Cabanel, Etablissement Français du Sang, Paris, France. Ethical committee permission was obtained for the use of buffy bags of healthy donors (N°12/EFS/079). B cells were isolated from PBMCs by positive selection using the human CD19 microbeads and monocytes were purified by using human CD14 microbeads. Monocytes (0.5 × 10 6 cells per ml) were cultured in the presence of granulocyte macrophage colony-stimulating factor (GM-CSF; 1,000 IU per 10 6 cells) and IL-4 (500 IU per 10 6 cells) (both cytokines from Miltenyi Biotec) for 5–7 days to obtain immature monocyte-derived DCs. CD4 + T cells were either selected positively by CD4 microbeads or by negative selection using CD4 + T-cell isolation kit II. Further, from the negatively selected T cells, naive CD4 + T cells were isolated by selectively depleting CD45RO + T cells by using CD45RO microbeads. The purity of the separated cells was >95% in all the populations. B-cell stimulation Freshly isolated B cells were used as ‘resting B cells’ for co-culture with DCs. For pre-activation, B cells (0.5 × 10 6 cells per ml) seeded in U-bottom 96-well plates were stimulated via BCR using F(ab′) 2 of goat anti-human IgM (10 μg ml −1 ) or with CD40-mediated signalling using agonistic anti-human CD40 monoclonal antibody (mAb; mouse IgG2B clone 82111, R&D Systems, Lille, France; 5 μg ml −1 ) or with BCR+CD40 or recombinant CD40 ligand (CD40L, R&D Systems; 5 μg ml −1 )+IL-4 (500 U ml −1 ) for 48 h to obtain ‘activated B cells’. The agonistic nature of anti-CD40 antibodies was confirmed by various approaches. Anti-CD40 mAbs induced clustering, proliferation and activation of B cells. In a synergistic manner, anti-CD40 agonistic antibodies enhanced B-cell activation and proliferation induced by BCR signalling. Moreover, B cells stimulated with anti-CD40 agonistic antibodies induced significant proliferation of allogeneic T cells. Supernatants from activated B-cell cultures were collected and centrifuged at 10,000 r.p.m. for 10 min to remove cellular debris. Before co-culture with immature DCs, both resting and pre-activated B cells were treated with mitomycin C (50 μg ml −1 ; Sigma-Aldrich, Saint-Quentin Fallavier, France) or paraformaldehyde fixed (1% in PBS for 30 min at 4 °C) and washed thoroughly to generate mitotically inactive cells to keep the B-cell number constant in B cell–DC co-culture systems. B cell–DC co-cultures Immature monocyte-derived DCs (0.1 × 10 6 cells per 200 μl per well) with GM-CSF and IL-4 were cultured either alone or with B cells (resting or pre-activated) at the ratio of 1:1 in U-bottom 96-well plates for 48 h. In some experiments, DCs were stimulated with recombinant human TSLP (20 ng per 0.1 × 10 6 cells, R&D Systems). For transwell experiments, B cells and DCs were kept separated by a 0.4-μm membrane. DCs (0.5 × 10 6 in 600 μl) were placed in the lower chamber of the transwell plate and pre-activated B cells (0.5 × 10 6 in 100 μl) in the upper chamber. For the stimulation of DCs using supernatant from activated B cells, immature DCs (0.1 × 10 6 cells per 250 μl total volume per well) were cultured in GM-CSF and IL-4 alone, or with supernatant from activated B cells (200 μl per well). In some experiments, resting B cells were directly stimulated in DC–B cell co-culture by using F(ab′) 2 of goat anti-human IgM (10 μg ml −1 ). In these experiments, the role of various surface molecules in contact-dependent induction of maturation of DCs by activated B cells was explored by employing blocking mAbs to anti-CD69 (10 μg ml −1 ), anti-TACI (10 μg ml −1 ), anti-CD54 (10 μg ml −1 ), anti-BAFF-R (10 μg ml −1 ) and anti-CD11a (10 μg ml −1 ), or mouse IgG isotype control antibodies (all from R&D systems). DC–T cell co-culture and mixed lymphocyte reaction Following 48 h of B cell–DC co-culture, B cells were depleted using CD20 microbeads and B-cell-depleted DCs were used for the co-culture with T cells. The purity of DCs following B-cell depletion was up to 98%. For mixed lymphocyte reaction, graded doses of B-cell-depleted DCs were co-cultured in U-bottom 96-well plate with allogeneic total CD4 + T cells (0.05 × 10 6 per well per 200 μl) in complete RPMI-1640 medium supplemented with 10% human AB serum. After 4 days of culture, 50 μl of supernatants were collected from each well before pulsing cells with 1 μCi (0.037 MBq) [ 3 H]thymidine overnight to quantify T-cell proliferation. Radioactive incorporation was measured by standard liquid scintillation counting and results were expressed as counts per minute. For analysing DC-mediated T-cell polarization, DCs were seeded with CD45RO − naive Th cells (0.1 × 10 6 per well per 200 μl) in the ratio of 1:20 in U-bottom 96-well plate. For blocking experiments, B-cell-depleted DCs were pre-incubated with either isotype control antibody or anti-OX40L (10 μg ml −1 ) for 30 min before co-culture with T cells. Following 6 days, cell-free supernatants were collected to analyse various T-cell cytokines by enzyme-linked immunosorbent assay. Cells were split into two parts and one part of cells was stained for surface molecules and intracellular T-cell transcription factor. The other part was restimulated for intracellular cytokine staining. Cytokine and chemokine assay BD Cytokine Bead Array (CBA) kits (BD Biosciences, Paris, France) for human inflammatory cytokines (IL-1β, CXCL8/IL-8, TNF-α, IL-6, IL-10 and IL-12p70) and human Th1/Th2 cytokines (IL-2, IL-4, IL-5, IL-10, TNF-α and IFN-γ) were used to determine the cytokine levels in the supernatants. IL-33 and IL-17A, and chemokines CCL3, CCL4, CCL17, CCL18, CCL22, CXCL9, CXCL10 and CXCL16 were quantified using DuoSet ELISA kit (R&D Systems). IL-13, IL-17F and IL-22 were analysed using ELISA Ready-SET-Go kits (eBioscience, Paris, France). IL-21 was determined using ELISA MAX Deluxe Sets (BioLegend, San Diego, USA). Flow cytometry The following fluorochrome-conjugated antibodies were used at a dilution of 1 in 50. BD Biosciences: fluorescein isothiocyanate-conjugated antibodies to CD1a, CD86, HLA-DR, CD71, IFN-γ and Foxp3; PE-conjugated antibodies to CD25, CD83, CD80, TACI and IL-4; APC-conjugated antibodies to CD19, CD20 and CD40L; Pacific blue-conjugated antibodies to CD4 and CD20; anti-CD69-APC-Cy7; anti-CCR4-PE-Cy7; and anti-CXCR3-AF700. Antibodies from eBioscience included CD40-APC, CD1a-Pacific Blue, CXCR5-PE, IL-6-APC, IL-17A-PE, TACI-PE, BAFF-R-fluorescein isothiocyanate, TNF-α-AF700, IFN-γ-APC-efluor 780, GATA3-PerCP-eFluor 710, T-bet-PE-Cy7, RORC-APC and Foxp3-APC. In addition, antibodies to CD3 (BV605), helios (22F6), CD11c (BV711), CD20 (BV650), CD27 (PE-Cy7), CD80 (BV605), CD206 (APC-Cy7), DC-SIGN (PE-Cy7), CCR7 (BV711), CCR6 (BV605), Ki-67 (BV711), IL-2 (BV650), IL-4 (PE), IL-17A (BV421), OX-40L (PE) and IL-8 (PerCP-Cy5.5) from BioLegend and anti-CD40-PE from Beckman Coulter (Villepinte, France) were also used. Cells for surface staining were suspended in 10% FCS/PBS and antibodies against surface molecules were added at pre-determined concentration and incubated for 20 min at 4 °C. After washing, cells were fixed with BD Fix buffer and washed before analysis on flow cytometer. The data are presented as percentage of cells positive for indicated molecules or mean fluorescence intensities (MFI) of their expression. For intracellular staining, DC–T cell co-cultures were stimulated with phorbol myristate acetate (50 ng ml −1 ; Sigma-Aldrich) and ionomycin (500 ng ml −1 ; Sigma-Aldrich) at 37 °C for 5 h in the presence of BD golgistop and BD golgiplug during the last 4 h. Following surface staining, cells were fixed and permeabilized (Foxp3 Fixation/Permeabilization kit, eBioscience) according to the manufacturer’s instructions, and incubated at room temperature with fluorescence-conjugated mAbs. Cells were acquired on LSRII and processed with FACS DIVA software (BD Biosciences) and analysed by Flowjo. IgE production by B cells CD19 + B cells were isolated from PBMC and were cultured in RPMI-1640–10% FCS either alone (0.02 × 10 6 cells per well per 200 μl) in U-bottomed 96-well plates or with T cells at 1:2.5 ratio for 12 days. Cell-free culture supernatants were collected and quantity of IgE was measured by enzyme-linked immunosorbent assay (Bethyl Laboratories, Euromedex, Soufflweyersheim, France). Statistical analysis One-way analysis of variance (repeated measures with Tukey’s multiple comparison test) was used to determine the statistical significance of the data. P <0.05 was considered significant. How to cite this article: Maddur, M. S. et al. Human B cells induce dendritic cell maturation and favour Th2 polarization by inducing OX-40 ligand. Nat. Commun. 5:4092 doi: 10.1038/ncomms5092 (2014).